Integrating a redox-coupled dye-sensitized photoelectrode into a lithium–oxygen battery for photoassisted charging With a high theoretical specific energy, the non-aqueous rechargeable lithium–oxygen battery is a promising next-generation energy storage technique. However, the large charging overpotential remains a challenge due to the difficulty in electrochemically oxidizing the insulating lithium peroxide. Recently, a redox shuttle has been introduced into the electrolyte to chemically oxidize lithium peroxide. Here, we report the use of a triiodide/iodide redox shuttle to couple a built-in dye-sensitized titanium dioxide photoelectrode with the oxygen electrode for the photoassisted charging of a lithium–oxygen battery. On charging under illumination, triiodide ions are generated on the photoelectrode, and subsequently oxidize lithium peroxide. Due to the contribution of the photovoltage, the charging overpotential is greatly reduced. The use of a redox shuttle to couple a photoelectrode and an oxygen electrode offers a unique strategy to address the overpotential issue of non-aqueous lithium–oxygen batteries and also a distinct approach for integrating solar cells and batteries. The lithium–oxygen (Li–O 2 ) batteries are recently attracting increasing research attention because of their higher specific energy density compared with conventional Li-ion batteries [1] , [2] , [3] , [4] , [5] , [6] , [7] . In a typical non-aqueous rechargeable Li–O 2 battery, lithium peroxide (Li 2 O 2 ) is the discharging product formed on the oxygen electrode surface and is oxidized back to O 2 and Li + in a following charging process. However, the insulating property of bulk Li 2 O 2 and the sluggish kinetics of the Li 2 O 2 oxidation reaction make it difficult to electrochemically decompose Li 2 O 2 efficiently [8] . This leads to a severe charging overpotential issue, which causes not only a very low battery round-trip efficiency, but also the decompositions of the oxygen electrode and electrolyte [3] , [4] , [7] , [9] . Recently, redox shuttles, such as tetrathiafulvalene (TTF + /TTF), have been introduced in the battery electrolyte to address this poor charge transport issue [10] , [11] , [12] , [13] , [14] . During the charging process, the reduced form of the redox shuttle, M red , is first converted to M ox on the oxygen electrode, which in turn oxidizes the Li 2 O 2 . By efficiently shuttling charges between Li 2 O 2 particles and the oxygen electrode surface, it facilitates the oxidation of Li 2 O 2 and therefore reduces the overpotential [13] , [14] . In this work, we introduce the approach of using a redox shuttle to couple a photoelectrode with the oxygen electrode in non-aqueous Li–O 2 batteries, which enables the photoassisted charging process. The photovoltage generated on the photoelectrode compensates the battery’s charging voltage. By utilizing solar energy, the device can be charged with a ‘negative’ overpotential, which is otherwise thermodynamically impossible. This concept of ‘photoassisted charging process’ offers a novel strategy to address the overpotential issue of non-aqueous Li–O 2 batteries and also a distinct approach for integrating solar cells and batteries [15] , [16] , [17] , [18] . 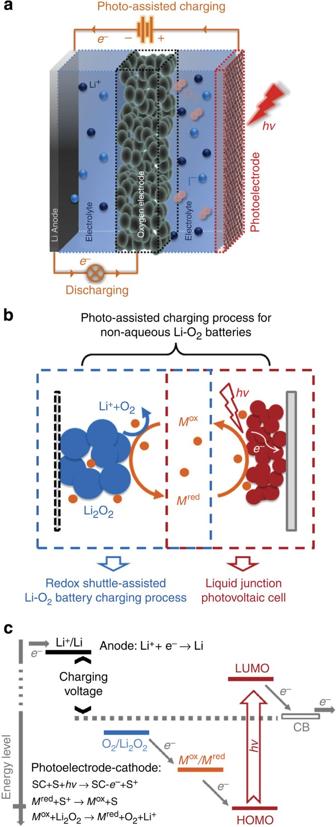Figure 1: The photoassisted charging process of the solar battery. (a) The scheme of a three-electrode solar battery: The solar battery consists of a Li anode, an oxygen electrode and a photoelectrode. On charging, the photoelectrode and Li anode are connected to the outside circuit; while on discharging, the oxygen electrode and Li anode are connected to the outside circuit. (b) The proposed photoelectrochemical mechanism of the photoassisted charging process: on charging under illumination, the redox shuttle in its reduced form (Mred) first gets oxidized toMoxon the photoelectrode and then diffuses to the Li2O2particles that are deposited on the oxygen electrode. By oxidizing the Li2O2into O2and Li+, theMoxis reduced back toMred. (c) The energy diagram of a solar battery which integrates a dye-sensitized semiconductor photoelectrode. (‘SC’ stands for semiconductor and ‘S’ stands for sensitizer.) The photoassisted charging voltage is determined by the energy difference between the Li+/Li redox potential and the quasi-Fermi level of electrons in the semiconductor electrode (at best close to its conduction band (CB) edge.) General design of the solar battery Figure 1a shows the structure of the device, named as solar battery, in this work. It consists of three electrodes: a Li-metal anode, an oxygen electrode made from carbon paper and a photoelectrode. The discharging process remains the same as that of a conventional Li–O 2 battery with the formation of Li 2 O 2 at the oxygen electrode. The charging process is, however, different. The charging voltage is applied on the Li-metal anode and the photoelectrode. Under illumination, a photoelectrochemical oxidation occurs on the photoelectrode first, converting M red into M ox , which in turn diffuses to the oxygen electrode and oxidizes Li 2 O 2 ( Fig. 1b ). In this photoassisted charging process, the photovoltage generated on the photoelectrode is utilized to compensate the required charging potential. Figure 1: The photoassisted charging process of the solar battery. ( a ) The scheme of a three-electrode solar battery: The solar battery consists of a Li anode, an oxygen electrode and a photoelectrode. On charging, the photoelectrode and Li anode are connected to the outside circuit; while on discharging, the oxygen electrode and Li anode are connected to the outside circuit. ( b ) The proposed photoelectrochemical mechanism of the photoassisted charging process: on charging under illumination, the redox shuttle in its reduced form ( M red ) first gets oxidized to M ox on the photoelectrode and then diffuses to the Li 2 O 2 particles that are deposited on the oxygen electrode. By oxidizing the Li 2 O 2 into O 2 and Li + , the M ox is reduced back to M red . ( c ) The energy diagram of a solar battery which integrates a dye-sensitized semiconductor photoelectrode. (‘SC’ stands for semiconductor and ‘S’ stands for sensitizer.) The photoassisted charging voltage is determined by the energy difference between the Li + /Li redox potential and the quasi-Fermi level of electrons in the semiconductor electrode (at best close to its conduction band (CB) edge.) Full size image In general, either a dye-sensitized photoelectrode or a semiconductor-electrolyte junction can be applied in the solar battery ( Fig. 1c and Supplementary Fig. 1 ) [19] , [20] . Figure 1c shows the energy diagram of the solar battery based on a dye-sensitized TiO 2 photoelectrode [20] , [21] , [22] , [23] , as a demonstration of the concept. On charging under illumination, the photoexcited dye molecules inject electrons into the conduction band of TiO 2 and are regenerated by oxidizing the M red to M ox . The formed M ox species subsequently diffuse to the oxygen electrode, oxidize the solid Li 2 O 2 to O 2 and are reduced back to complete a full redox cycle. The charging voltage equals the energy difference between the redox potential of the Li + /Li couple and the quasi-Fermi level of electrons in the TiO 2 photoelectrode (which is at best close to the conduction band minimum of TiO 2 , ~+2.6 V versus Li + /Li [22] , [23] , all potentials in this manuscript refer to the Li + /Li redox) ( Fig. 1c ). Therefore, we expect that the solar battery has a lower charging voltage than any other conventional non-aqueous Li–O 2 batteries, which have their charging voltage limitation as 2.96 V (that is, the redox potential of O 2 /Li 2 O 2 ) controlled by thermodynamics. The I 3 − /I − redox couple for non-aqueous Li–O 2 batteries For dye-sensitized TiO 2 solar cells, the triiodide/iodide (I 3 − /I − ) redox couple is a benchmark electrolyte for the dye regeneration [24] . Despite being mentioned in a patent [12] and a very recent publication [14] , not much attention has been placed on utilizing I 3 − /I − redox couple for non-aqueous Li–O 2 batteries. Therefore, we started with investigating the I 3 − /I − couple as a redox shuttle for Li–O 2 batteries. The cyclic voltammetry (CV) reveals that the redox potential of I 3 − /I − couple in 1 M LiClO 4 /dimethylsulfoxide (DMSO) solution is about +3.55 V ( Supplementary Fig. 2 ), consistent with earlier study [24] . Hence, the oxidization of Li 2 O 2 by I 3 − is considered to be thermodynamically favourable with a driving force of 0.59 V (3.55 V−2.96 V=0.59 V). Meanwhile, the CV shape of I 3 − /I − redox kept almost identical when the argon atmosphere was replaced by oxygen, indicating its good stability. Li–O 2 batteries were then assembled with surface pretreated Li-metal foil as the anode [25] , commercial P50 carbon paper as the oxygen electrode and a piece of glassy fibre separator [9] , [26] , [27] in between. A solution of 0.1 M LiI and 1 M LiClO 4 in DMSO was used as the electrolyte. (For experimental details, see Methods). The batteries were cycled under one atmosphere of pure O 2 . A comparison of discharge–charge curves between batteries with and without the redox shuttle is shown in Fig. 2a . At a current flow of 0.16 mA cm −2 , on charging, the battery with LiI showed a voltage plateau at about 3.5 V, matching well with the I 3 − /I − redox potential. In contrast, the battery without LiI in the electrolyte had its charging voltage quickly climbing up to above 4.0 V. Moreover, batteries with LiI could be charged with a voltage around 3.6 V even at a current flow as high as 0.47 mA cm −2 ( Supplementary Fig. 3a ). Their cyclability was also evaluated. As shown in Fig. 2b , the batteries could be cycled at 0.16 mA cm −1 for at least 25 cycles with only small performance decay. More detailed analysis and discussion of the battery performance are presented in the Supplementary Information ( Supplementary Figs 3 and 4 ). 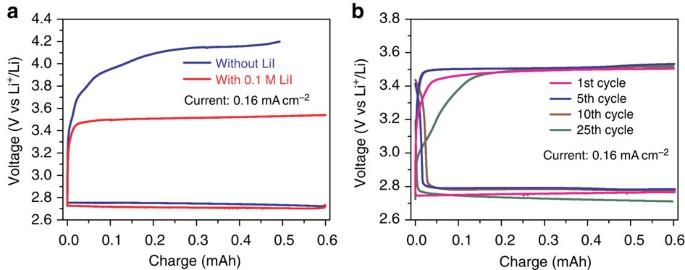Figure 2: Electrochemical characterizations of Li–O2batteries with and without the LiI redox shuttle. (a). The first-cycle discharge–charge curve of a Li–O2battery with and without LiI redox shuttle at a current density of 0.16 mA cm−2. The electrolyte is 1.0 M LiClO4in DMSO solvent. (b). The discharge–charge curves of a Li–O2battery with 0.1 M LiI, at the 1st, 5th, 10th and 25th cycle. The current density is 0.16 mA cm−2and the electrolyte is 1.0 M LiClO4, 0.1 M LiI in DMSO solvent. The tests are replicated for more than five times. Figure 2: Electrochemical characterizations of Li–O 2 batteries with and without the LiI redox shuttle. ( a ). The first-cycle discharge–charge curve of a Li–O 2 battery with and without LiI redox shuttle at a current density of 0.16 mA cm −2 . The electrolyte is 1.0 M LiClO 4 in DMSO solvent. ( b ). The discharge–charge curves of a Li–O 2 battery with 0.1 M LiI, at the 1st, 5th, 10th and 25th cycle. The current density is 0.16 mA cm −2 and the electrolyte is 1.0 M LiClO 4 , 0.1 M LiI in DMSO solvent. The tests are replicated for more than five times. Full size image The dye-sensitized TiO 2 -based solar battery With the I 3 − /I − couple demonstrated as an efficient redox shuttle for Li–O 2 batteries, we then consider the structural details of a solar battery. The photoelectrode was a titanium metal gauze decorated with rutile-phase TiO 2 nanorods ( Fig. 3a and Supplementary Fig. 5 ) and sensitized by the Ruthenizer 535 bis-TBA dye (N719) (ref. 28 ). The open structure of the wire gauze allows the diffusion of oxygen through the photoelectrode to the oxygen electrode. To test the photochemical activity of this dye-sensitized TiO 2 electrode, a solar cell was fabricated. Its photocurrent–voltage curve shows that such a photoelectrode is capable of generating an open-circuit voltage of about 0.73 V under illumination ( Fig. 3b ). In such a dye-sensitized TiO 2 solar cell, the dye regeneration reaction, which eventually yields I 3 − from I − , is an ‘ in situ ’ process with the time constant on micron-second scale [24] , [29] . Meanwhile, the robustness of the I 3 − in oxidizing Li 2 O 2 has also been demonstrated in the battery tests. Therefore, we consider the I 3 − /I − couple as an efficient charge transfer shuttle for transporting electrons between the photoelectrode and oxygen electrode: 2Dye + +3I − →2Dye+I 3 − (that is, the dye reduction), I 3 − +Li 2 O 2 →3I − +2Li + +O 2 (that is, the Li 2 O 2 oxidation). 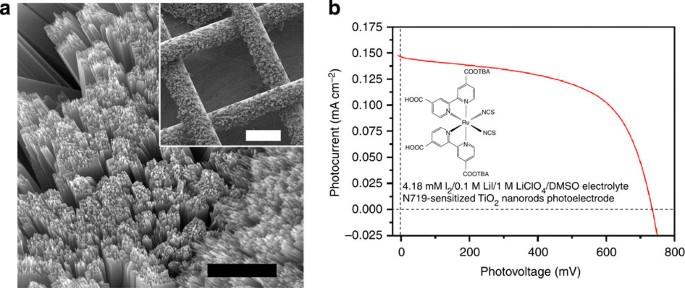Figure 3: Characterizations of the dye-sensitized TiO2photoelectrode. (a) Representative scanning electron microscopy images for the TiO2photoelectrode: the rutile-phase TiO2nanorods were hydrothermally grown on the Ti gauze. (scale bar, 1 μm; scale bar of the inset image, 100 μm). The open structure of the gauze, shown as the inset, allows the diffusion of oxygen to the oxygen electrode for the Li2O2formation; (b). The photocurrent–voltage (J–V) curve of a dye-sensitize solar cell based on this TiO2photoelectrode, with the inset as the molecular structure of N719 sensitizer. TheJ–Vcurve shows that this nanorod TiO2@ Ti gauze photoelectrode could work efficiently by providing an open-circuit voltage ~0.73 V. Figure 3: Characterizations of the dye-sensitized TiO 2 photoelectrode. ( a ) Representative scanning electron microscopy images for the TiO 2 photoelectrode: the rutile-phase TiO 2 nanorods were hydrothermally grown on the Ti gauze. (scale bar, 1 μm; scale bar of the inset image, 100 μm). The open structure of the gauze, shown as the inset, allows the diffusion of oxygen to the oxygen electrode for the Li 2 O 2 formation; ( b ). The photocurrent–voltage ( J – V ) curve of a dye-sensitize solar cell based on this TiO 2 photoelectrode, with the inset as the molecular structure of N719 sensitizer. The J – V curve shows that this nanorod TiO 2 @ Ti gauze photoelectrode could work efficiently by providing an open-circuit voltage ~0.73 V. Full size image The comparison of charging curves of a simple Li–O 2 battery, a Li–O 2 battery with the I 3 − /I − redox shuttle and a solar battery is shown in Fig. 4a,b , at different current densities. Apparently, the addition of I 3 − /I − redox shuttle has significantly reduced the charging voltage. It was further reduced with the incorporation of the photoelectrode: the solar battery charging voltage was recorded as 2.72 and 2.83 V at 0.016 and 0.032 mA cm −2 , respectively. Considering the small energy difference between the TiO 2 conduction band minimum (that is, ~+2.6 V) and quasi-Fermi level of electrons in the photoelectrode, we conclude that the results agree well with theoretical predictions. It is also noticeable that the charging voltage is lower than the O 2 /Li 2 O 2 redox potential (that is, +2.96 V), which is thermodynamically impossible without the solar energy input. Once illumination was removed, the voltage increased immediately, indicating the photovoltage no longer existing to compensate the charging voltage of the solar battery. ( Supplementary Fig. 6 ) Such a ‘light-response’ behaviour further supports our proposed working mechanism for this photoassisted charging process. 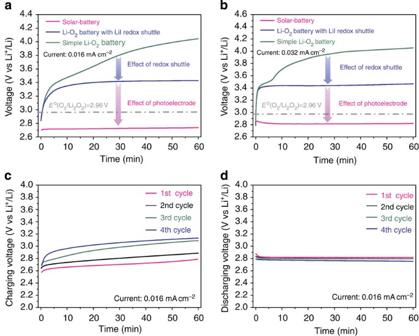Figure 4: Electrochemical characterizations of the solar battery. The charging curves of a simple Li–O2battery, the Li–O2battery with LiI redox shuttle and the solar battery at a current density of (a) 0.016 mA cm−2and (b) 0.032 mA cm−2. The LiI redox shuttle and photoelectrode significantly reduces the battery charging voltage. The solar battery performance of the first four cycles with a current density of 0.016 mA cm−2: (c) the charging curves and (d) the discharging curves. The charging curves for the first four cycles show a gradual voltage increasing, which is attributed to the decomposition of the N719 sensitizer under the strong oxidation environment. The tests are replicated for more than three times. Figure 4: Electrochemical characterizations of the solar battery. The charging curves of a simple Li–O 2 battery, the Li–O 2 battery with LiI redox shuttle and the solar battery at a current density of ( a ) 0.016 mA cm −2 and ( b ) 0.032 mA cm −2 . The LiI redox shuttle and photoelectrode significantly reduces the battery charging voltage. The solar battery performance of the first four cycles with a current density of 0.016 mA cm −2 : ( c ) the charging curves and ( d ) the discharging curves. The charging curves for the first four cycles show a gradual voltage increasing, which is attributed to the decomposition of the N719 sensitizer under the strong oxidation environment. The tests are replicated for more than three times. Full size image To evaluate the coulombic efficiency of this photoassisted charging process, the amount of Li 2 O 2 on the oxygen electrode before and after the charging process was quantified. It is based on the fast and quantitative reaction: [TiO] 2+ SO 4 2− +Li 2 O 2 +2H + →[TiO 2 ] 2+ SO 4 2− +2Li + +H 2 O (ref. 30 ). The formed [TiO 2 ]SO 4 complex has a characteristic absorption peak at 405 nm. Therefore, the amount of Li 2 O 2 involved in the reaction can be calculated based on the absorbance data. Experimentally, before the photoassisted charging process, 1.76 μmol Li 2 O 2 was deposited on the oxygen electrode by a previous discharging process. After a charging process with 3.60 μmol electrons passing through, no detectable Li 2 O 2 was left ( Supplementary Fig. 7 ). The molar ratio of the oxidized Li 2 O 2 to the electrons passed through is 1:2.05, matching well with the theoretical 1:2 mol ratio (Li 2 O 2 : e − ). This result, together with the Raman spectra ( Supplementary Fig. 8 ), proves that the Li 2 O 2 has been efficiently oxidized by the I 3 − that generated on the photoelectrode. The solar battery was rechargeable ( Fig. 4c,d ), however, with a performance decay as cycling went on. By checking the electrodes before and after the solar battery cycling via X-ray photoelectron microscopy (XPS), we attribute this to the gradual decomposition of N719 dye molecules under the strong oxidizing environment ( Supplementary Figs 9–11 ). Hence, improving the stability of photoelectrode is essential. This issue can be solved by replacing the dye-sensitized TiO 2 with other more stable photoelectrodes. In fact, our preliminary results of the haematite (that is, α-Fe 2 O 3 ) photoelectrode based solar battery have shown that a single semiconductor–liquid junction photoelectrode also works efficiently and presents a remarkably better stability. A more detailed discussion of the haematite-based solar battery is presented in the Supplementary Information ; ( Supplementary Fig. 12 ). Besides solving the stability issue, the success on haematite-based solar battery further proves that the concept of photoassisted charging process has its generic impact on addressing the charging overpotential issue for Li–O 2 batteries. More work on extending this concept to a large library of photoelectrode materials, such as haematite, doped TiO 2 , BiVO 4 and so on, is currently undergoing. In conclusion, a photoassisted charging process for the non-aqueous Li–O 2 battery has been demonstrated on a solar battery, which integrates a dye-sensitized TiO 2 photoelectrode with the oxygen electrode via the linkage of the triiodide/iodide redox shuttle. On charging under illumination, the photoelectrode generates triiodide ions that subsequently diffuse to the oxygen electrode surface and oxidize Li 2 O 2 . The photovoltage generated on the TiO 2 photoelectrode compensates the battery’s charging voltage. By utilizing solar energy, the device can be charged with a ‘negative’ overpotential, which is otherwise thermodynamically impossible. The proposed photoassisted charging process has been proved to be efficient. The performance of the solar battery will be further improved by optimizing the device configuration and exploring more stable photoelectrode materials. With this concept demonstrated, our work provides a novel and generic strategy to address issues of low energy efficiency and side reactions brought by the high charging overpotential for non-aqueous Li–O 2 batteries. Furthermore, by using a redox shuttle to couple a photoelectrode and a battery into one device, this work also suggests a distinct approach for integrating solar cells and batteries, which represents an important direction for the future applications in solar energy conversion and storage. Battery and solar battery assembly All devices were assembled in an argon gas-filled glovebox. For Li–O 2 batteries: the Li foil (0.75 mm thick, 99.9%, Alfa-Aser) was pretreated in 1 M lithium perchlorate (LiClO 4 , 99.99%, Sigma-Aldrich) of propylene carbonate (PC, 99.7%, Sigma-Aldrich) solution for three days before used as the anode [9] . A piece of commercial P50 carbon paper (0.25 mm thick, ~3.5 mg, AvCarb) and a piece of stainless steel gauze as the current collector (100-mesh, 0.25 mm thick, Fisher-Scientific) were stacked and used as the oxygen electrode. A piece of glassy fibre (0.6 mm thick, Whatman), saturated by the electrolyte as a solution of 0.1 M LiClO 4 in DMSO (99.9%, Sigma-Aldrich), was used as the separator. For the batteries with I 3 − /I − redox shuttle, 0.1 M LiI (99.9%, Sigma-Aldrich) was added in the electrolyte. The batteries were assembled as Swagelok cells with an O-ring sealing. One atmosphere of high pure O 2 was introduced to the oxygen electrode. For solar batteries, the anode and the oxygen electrode were the same as for Li–O 2 batteries. For the photoelectode, TiO 2 nanorods were hydrothermally grown on a piece of Ti gauze (80-mesh, Fisher-Scientific) based on a modified recipe [31] . Briefly, the Ti gauze (~10 mg) was first heated at 500 °C for 30 min in air to get a dense TiO 2 coating layer. Then the gauze was placed in an aqueous solution (14 ml) of 225 μl titanium chloride (99.0%, Sigma-Aldrich) and 0.7 ml HCl (~37%, Fisher-Scientific) and hydrothermally heated at 170 °C for 10 h. After reaction, the TiO 2 nanorod-decorated Ti gauze was washed with water, sintered at 450 °C for 30 min and then sensitized with N719 dye molecules (Solaronix). A piece of glassy fibre (0.35 mm thick, VWR) saturated with the 1.0 M LiClO 4 /0.1 M LiI/DMSO electrolyte was used to separate the oxygen electrode and photoelectrode. A fused silica window was O-ring sealed on the cell for allowing the illumination on the photoelectrode. For testing the solar cell, a sandwiched cell was made by a N719-sensitized TiO 2 photoelectrode, a platinum-coated fluorine-doped tin oxide glass counter electrode and an electrolyte as 4.18 mM I 2 , 0.1 M LiI and 1 M LiClO 4 in DMSO. Electrochemical and photoelectrochemical cell testing Li–O 2 batteries were tested using a Maccor testing station (model: 4304), within a voltage range between 2.0 and 4.2 V (versus Li + /Li), with discharge and charge current densities varying from 0.016 to 0.79 mA cm −2 . For solar batteries, the anode and the oxygen electrode were connected to the outside circuit for discharging, while for charging, the anode and the photoelectrode were connected to the outside circuit. A small-area class-B solar simulator (PV Measurements) was used for obtaining a 1.5 Sun AM 1.5 illumination for the solar battery and solar cell tests. CV studies for the I 3 − /I − redox couple were carried out on a Gamry potentiostat in a three-electrode configuration, with a glassy carbon working electrode (3 mm diameter), a platinum wire counter electrode and a Ag + /Ag non-aqueous reference electrode (10 mM AgNO 3 in acetonitrile, from CHI, Inc.). The electrolyte was a solution of 1 M LiClO 4 and 5 mM I 2 in DMSO. Either argon or oxygen gas was saturated in the electrolyte during the CV tests. The scan rate was 10 mV s −1 . Characterizations After battery and solar battery tests, the devices were disassembled in the glovebox. The oxygen electrodes were washed with 1,2-dimethoxyethane (Novolyte Tech) and the electrolyte was collected. The Raman spectra of discharged and charged carbon paper oxygen electrodes were collected on a microscope Raman spectrometer (inVia, Renishaw) with a 633-nm excitation wavelength (laser power: 6 mW), using an air-sensitive sample holder with a fused silica optical window. The attenuated total reflectance—Fourier transform infrared spectra of discharged and charged carbon paper oxygen electrodes were collected inside a glovebox on a Frontier FT-IR/FIR spectrometer (PerkinElmer) with a diamond window. The XPS analyses of the electrodes were performed on a Kratos Axis Ultra XPS with monochromatic Al X-ray source, at an operation voltage as 12 kV and a current as 10 mA. All the XPS samples were protected from the ambient atmosphere using an air-tight sample transfer module. The scanning electron microscopy (FEI/Philips Sirion Field Emission SEM) was used to obtain the morphology of the TiO 2 nanostructure for the photoelectrode and the discharging product on the oxygen electrode. The X-ray diffraction instrument (Cu Kα, Rigaku, Inc.) was used to determine the crystal phase of TiO 2 nanorods and the discharging product on the oxygen electrode. For the quantitative analysis of Li 2 O 2 amount, a calibration curve was first made by reacting different amounts of lithium peroxide with 2 ml ~15% wt titanium(IV) oxysulfate (TiOSO 4 )/sulfuric acid (H 2 SO 4 ) solution (99.99%, Sigma-Aldrich) (>100 magnitude excess to the Li 2 O 2 ) and measuring the absorbance of formed [TiO 2 ] 2+ at 405 nm with ultraviolet-visible (UV–vis) spectra on a Lambda 950 UV/Vis/NR spectrometer (PerkinElmer). Then, two parallel solar batteries were assembled and discharged with the same capacity. One was disassembled in the glovebox and the carbon paper oxygen electrode was reacted with 2 ml TiOSO 4 /H 2 SO 4 solution. The Li 2 O 2 amount was determined by UV–vis spectra. The other solar battery was charged under illumination with 3.60 μmol electron passing through. After charging, the oxygen electrode was also reacted with 2 ml TiOSO 4 /H 2 SO 4 solution and the Li 2 O 2 amount left was determined by UV–vis spectra. How to cite this article : Yu, M. et al . Integrating a redox-coupled dye-sensitized photoelectrode into a lithium–oxygen battery for photoassisted charging. Nat. Commun. 5:5111 doi: 10.1038/ncomms6111 (2014).